Gold-promoted structurally ordered intermetallic palladium cobalt nanoparticles for the oxygen reduction reaction Considerable efforts to make palladium and palladium alloys active catalysts and a possible replacement for platinum have had a marginal success. Here we report on a structurally ordered Au 10 Pd 40 Co 50 catalyst that exhibits comparable activity to conventional platinum catalysts in both acid and alkaline media. Electron microscopic techniques demonstrate that, at elevated temperatures, palladium cobalt nanoparticles undergo an atomic structural transition from core-shell to a rare intermetallic ordered structure with twin boundaries forming stable {111}, {110} and {100} facets via addition of gold atoms. The superior stability of this catalyst compared with platinum after 10,000 potential cycles in alkaline media is attributed to the atomic structural order of PdCo nanoparticles along with protective effect of clusters of gold atoms on the surface. This strategy of making ordered palladium intermetallic alloy nanoparticles can be used in diverse heterogeneous catalysis where particle size and structural stability matter. The search for new materials for the oxygen reduction reaction (ORR), a sluggish reaction that requires high Pt content hampering the large scale applications of electrochemical conversion and storage devices, such as fuel cells, Li-air batteries, certain electrolyser, has been challenging [1] , [2] . Key strategies to reduce Pt contents involve alloying Pt with other transition metal [3] , [4] , [5] , [6] , [7] , [8] , de-alloying non-precious metal to obtain a Pt rich shell [9] , [10] , [11] and core-shell-structured nanoparticles [12] , [13] , [14] , [15] . These approaches, to some degree, increase Pt utilization, but cannot fully solve the problem of Pt dependence. To substitute the active but expensive Pt-based ORR catalyst, recent advances have been made to develop low-cost alternatives such as metal-N complex on carbon matrixes [16] , [17] , perovskites [18] , spinel oxides [19] and carbon-based nanomaterials [20] . However, these current catalyst materials are still far from meeting the requirements of combined high catalytic activity, better durability and low cost [21] . Moreover, there is no single catalyst, rather than Pt-based catalyst, that can be as an electrocatalyst in both anion-exchange and proton-exchange membrane fuel cells. So, new strategies to develop efficient alternatives for Pt catalysts are still anticipated. The ORR at the cathode of the fuel cell varies with particle size, composition and structure of the electrocatalyst [22] , [23] . The benefits of size and structure manipulation of the nanoparticles have led us to develop a non-Pt-based catalyst that can be used both in alkaline and acidic media. The study of ORR on Pd-based electrodes in fuel cell has received less attention than on Pt due to the lower activity and stability of the former [24] , [25] . Moreover previous studies, with an exception of the intermetallic compound PdPb as support for a Pt monolayer [26] , have mainly been pursued on the Pd random alloy catalysts with various shapes and structures [27] , [28] , [29] , [30] , [31] , while no experimental studies have been focused on structurally ordered intermetallic PdCo nanocatalyst. This is due to concerns that PdCo do not form intermetallic phases in a nanometre range [32] , [33] during the high-temperature annealing, a general requirement to obtain ordered phases. However, using certain material composition and structure, ordered intermetallic phases can be obtained at nanometre ranges. Here, we address this challenge by demonstrating a simple method to make core-shell-structured PdCo nanoparticles that can be further transformed into ordered intermetallic phases by addition of Au atoms and subsequent annealing. The discovery of unusual ordering of PdCo atoms (3 × (times) and 2 × ) along the [111] direction in the AuPdCo nanoparticles with twin boundaries and with stable {111}, {110} and {100} facets is revealed using high-resolution transmission electron microscope (HRTEM) and scanning transmission electron microscope (STEM) coupled with electron energy-loss spectroscopy (EELS) and electron diffraction patterns (EDPs). To our knowledge, no prior evidence of such intermetallic phases in nanoparticles of PdCo alloy has previously been reported. These structurally ordered intermetallic AuPdCo nanoparticles tend to behave similar to Pt catalyst for ORR but more interestingly have much better stability than Pt in alkaline media. Furthermore, microscopic analyses of the catalyst shows that atomic ordering of the nanoparticles can significantly affect the catalytic activity. The increased activity and durability of the catalyst is accredited to multiple facets and the structural ordering observed in the nanoparticles. Structural properties of AuPdCo Initially, core-shell structures of AuPdCo nanoparticles that had an average diameter of 1 nm were obtained using the step-by-step chemical synthesis method (see Methods). The structures of the as-obtained core-shell nanoparticles were controlled by annealing at different temperatures under a flowing H 2 gas atmosphere. The nanoparticles tend to grow when annealed at 500 °C in H 2 for 30 min attaining an average diameter of 4 nm while maintaining their core-shell structure. As illustrated in Fig. 1a,b , the nanoparticles have a core-shell structure with AuPd atoms on the surface and Co in its core. We use the AuPdCo annealed at 500 °C sample as a reference for the disordered core-shell AuPdCo catalysts. The high angle annular dark-field images as shown in Fig. 1a (also Supplementary Fig. 1 ), whose contrast is directly related to atomic number Z (ref. 34 ), reveals that the intensity profile for Au and Pd is nearly depleted in the centre of the nanoparticle, whereas for Co it is enriched in the centre. EELS line-scan profile indicates the distribution of Au, Pd and Co components in a representative single nanoparticle, where the Pd shell thickness measured is around 0.9–1.2 nm and Au atoms are distributed on the surface. To attain an intermetallic ordered structuring of the nanoparticles, the as-obtained core-shell AuPdCo nanoparticles were annealed at 800 °C for 30 min, which reorganizes the PdCo atoms to a well-ordered structure with Au atoms on the surface. Because this behaviour of restructuring of core-shell PdCo nanoparticles to ordered intermetallic structure was not observed in the absences of Au atoms, we attribute this arrangement of PdCo atoms to the presence of Au atoms that may behave like a matrix or stabilizer shells [35] preventing the agglomeration of nanoparticles, meanwhile the temperature having a role in restructuring the PdCo atoms. 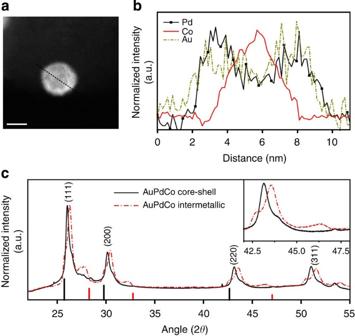Figure 1: STEM-EELS elemental line-scan profile and Synchrotron XRD patterns. (a,b) High angle annular dark-field-STEM image of a core-shell AuPdCo nanoparticle with its corresponding EELS line-scan profiles. Scale bar, 5 nm. (c) XRD patterns for core-shell and intermetallic AuPdCo nanoparticles. The black and red vertical lines indicate the (111), (200) and (220) peak positions of pure Pd and Co reflections, respectively. The inset shows the enlarged region of the AuPdCo (220) diffraction peaks. Figure 1: STEM-EELS elemental line-scan profile and Synchrotron XRD patterns. ( a , b ) High angle annular dark-field-STEM image of a core-shell AuPdCo nanoparticle with its corresponding EELS line-scan profiles. Scale bar, 5 nm. ( c ) XRD patterns for core-shell and intermetallic AuPdCo nanoparticles. The black and red vertical lines indicate the (111), (200) and (220) peak positions of pure Pd and Co reflections, respectively. The inset shows the enlarged region of the AuPdCo (220) diffraction peaks. Full size image Synchrotron X-ray diffraction (XRD) measurements as shown in Fig. 1c reveal some insights into the transformation of AuPdCo nanoparticles. The XRD patterns for both samples have four major diffraction peaks corresponding to (111), (200), (220) and (311) peaks that matches well to that expected from face-centered cubic (fcc) structure. Incorporation of Co into the Pd lattices shifts the peak positions to higher angles indicating lattice contraction. The intermetallic phase of the nanoparticles may have caused the peak for further contraction evident from the peak shifts to much higher angle than core-shell nanoparticles. The small shoulder-peak at 2 θ angles of 42.6° for (220) reflection (inset of Fig. 1c ) is due to the alloying effect of surface Au with Pd. Density functional theory studies have shown that Au atoms preferentially remain on the Pd surface by the segregation process [36] , [37] . The powder XRD patterns did not show the intermetallic phases of the nanoparticles. However, as discussed below, the electron microscopic analysis revealed the intermetallic structuring of the nanoparticles that has resulted in forming ordered Pd and Co planes ( Figs 2 and 3 and Supplementary Fig. 4 ). The small XRD peak positions at 2 θ angle of 46.3° near the pure Co-metal (220) reflections (inset of Fig. 1c ) may have been caused by the Co planes. The particle size calculated by Scherer equation using the (220) peaks was 6.8 nm and the lattice contraction was 0.9% more than the core-shell nanoparticles. 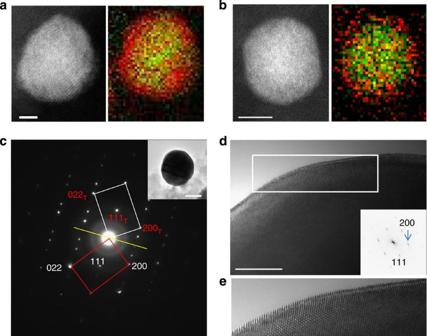Figure 2: STEM HRTEM and EDP along with two-dimensional EELS mapping. (a,b) Two-dimensional EELS mapping of Pd M-edge and Co L-edge (red-Pd atoms; green-Co atoms) from a single intermetallic AuPdCo nanoparticle. Scale bar, 2 and 5 nm, respectively. (c) EDP from a single particle as shown in the inset (scale bar, 50 nm) viewed along [01-1] direction. The EDP can be indexed as (01-1)* and (0–11)T* (subscript T denotes twin) patterns of fcc. The white and red rectangles outline the diffraction spots of the matrix and the twin whereas the yellow line shows the (111) twin plane. (d) HRTEM image from the top part of the particle inc. Scale bar, 10 nm. The inset is the diffractogram of the image. (e) Magnified image fromdshowing misfit between the shell and the core. Figure 2: STEM HRTEM and EDP along with two-dimensional EELS mapping. ( a , b ) Two-dimensional EELS mapping of Pd M-edge and Co L-edge (red-Pd atoms; green-Co atoms) from a single intermetallic AuPdCo nanoparticle. Scale bar, 2 and 5 nm, respectively. ( c ) EDP from a single particle as shown in the inset (scale bar, 50 nm) viewed along [01-1] direction. The EDP can be indexed as (01-1)* and (0–11) T * (subscript T denotes twin) patterns of fcc. The white and red rectangles outline the diffraction spots of the matrix and the twin whereas the yellow line shows the (111) twin plane. ( d ) HRTEM image from the top part of the particle in c . Scale bar, 10 nm. The inset is the diffractogram of the image. ( e ) Magnified image from d showing misfit between the shell and the core. 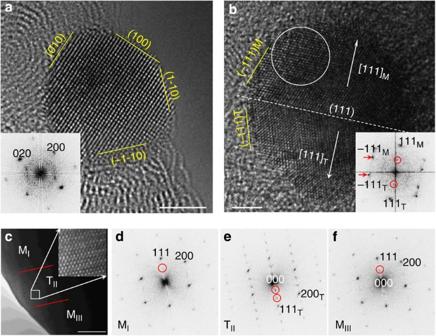Figure 3: Structural ordering of intermetallic AuPdCo nanoparticles. (a,b) HRTEM images from smaller nanoparticles viewed along [001] and [0–11] direction, respectively. Both scale bars, 3 nm. The diffractograms are embedded in the images. Ordering along [111] direction is visible inbas indicated by the white circle. Superlattice spots are also visible in the diffractogram as indicated by the red circles in the inset ofb. (c) HRTEM image from a large particle. The red lines incmark the twin boundaries. A close view (inset) shows the ordering along [111] direction. Scale bar, 10 nm. (d–f) The diffractograms from area MI, TIIand MIII, respectively. Superlattice spots are circled in red. Full size image Figure 3: Structural ordering of intermetallic AuPdCo nanoparticles. ( a , b ) HRTEM images from smaller nanoparticles viewed along [001] and [0–11] direction, respectively. Both scale bars, 3 nm. The diffractograms are embedded in the images. Ordering along [111] direction is visible in b as indicated by the white circle. Superlattice spots are also visible in the diffractogram as indicated by the red circles in the inset of b . ( c ) HRTEM image from a large particle. The red lines in c mark the twin boundaries. A close view (inset) shows the ordering along [111] direction. Scale bar, 10 nm. ( d – f ) The diffractograms from area M I , T II and M III , respectively. Superlattice spots are circled in red. Full size image Ordered intermetallic AuPdCo To understand the microstructure of intermetallic AuPdCo nanoparticles, bright field TEM images along with EELS two-dimensional imaging were performed. The images revealed that generally the particles were spherical with an average diameter of 6.7 nm ( Supplementary Fig. 2 ), which corresponds well to the value we determined in the XRD experiments. We found few large particles varying in size between 20- to 90-nm, while most particles (>~90%) were between 3- and 10-nm. The EELS mapping of Pd (M-edge) and Co (L-edge) from a single representative nanoparticle are shown in Fig. 2a,b , indicating an overall homogeneous distribution of Pd and Co atoms. Figure 2c shows a TEM image of a single large particle (inset) along with its EDP respectively viewed along the [01-1] direction. The EDP was indexed as fcc with lattice parameter of ~0.38 nm with (111) twin planes as shown by the diffraction spots of the matrix and the twin. To have a better insight to the arrangement of the atoms in the particle, a cropped high-resolution TEM (HRTEM) image from the top part of the particle is shown in Fig. 2d along with the diffractogram of the image in the inset. The HRTEM image in Fig. 2d is rotated about 49° with respect to the EDP as shown in Fig. 2c due to the magnetic lens in the microscope. When the HRTEM image is magnified as shown in Fig. 2e , the arrangement of atoms at the shell shows a misfit between the shell and the core demonstrating a PdAu alloy shell on the intermetallic arranged PdCo atoms ( Supplementary Fig. 2 ). The ordered intermetallic structure of the AuPdCo nanoparticles was often observed along [111] direction as shown in Fig. 3 , viewed along the [001] and the [0–11] zone axis. We can determine the intermetallic structure of the AuPdCo nanoparticles by selected-area electron diffraction patterns and HRTEM. The HRTEM from smaller particles ( Fig. 3a,b ) clearly show the {100}, {110} and {111} facets. The (111) reflection twins are present in smaller particles as shown in Fig. 3b , which also reveals the ordering along [111] direction. The superlattice spots can be identified from smaller particles as shown in the embedded diffractogram ( Fig. 3b ) though they are very weak. These spots could be easily identified from larger nanoparticles (50 nm) as shown in Fig. 3d–f . The (111) twinned boundaries (area T II ) as indicated by the red lines in Fig. 3c when magnified, clearly shows the ordering of atoms along the [111] direction. The diffractograms from area M I , T II and M III are shown in Fig. 3d–f , respectively. Two superlattice spots (marked by the circles) between 000 and 111 T in Fig. 3e was observed, confirming ordering along [111] direction. In fcc structure, normally Pd and Co randomly occupy at (111) planes ( Supplementary Fig. 4a ). The ordering occurs when Pd occupies in one (111) plane, while Co occupies in the other two planes (3 × (times) ordering), as shown in the simulated HRTEM ( Supplementary Fig. 4b ). The simulated HRTEM image and diffractogram based on the structure model are in good agreement with the experiments ( Fig. 3e ). This ordering of Pd and Co along [111] direction reduces the fcc symmetry (Fm-3m) to a primitive trigonal symmetry (P-3m, a~0.266 nm and c~0.651 nm). A different type of ordering of PdCo atoms was observed in the diffractograms from area M I and M III . Only one superlattice spot was observed between 000 and 111(marked by the circles) in the diffractograms, indicating ordering along the [111] direction. This kind of ordering occurs when Pd and Co atoms alternately stack (2 × ordering) along [111] direction. The simulated HRTEM image and diffractogram ( Supplementary Fig. 4c ) matches the observations from area M I and M III very well. The observed ordering along [111] direction reduces the fcc symmetry to rhombohedral symmetry (R-3m, a~0.266 nm and c~1.303 nm). Multiple low-index facets and superlattice spots of the structurally ordered AuPdCo nanoparticles were also viewed from other particles along the [0–11] zone axis as shown in Fig. 4 . The HRTEM image in Fig. 4b clearly shows the twin boundaries and the smooth {111}, {110} and {100} facets of the particle. The EDP was indexed as fcc with lattice parameter of 0.376 nm with (111) twins. The diffractograms from M I and M II are shown in Fig. 4e,d , respectively with weak superlattice spots in M I . Views along [0–11] and [001] direction from other nanoparticles ( Supplementary Fig. 3 ) show the ordered structure of the atoms along with antiphase domains, twin and facets. On the basis of the HRTEM images along with the appearance of superlattice spots in diffractograms that agree well with the diffractogram simulations ( Supplementary Fig. 4 ), we confirm that majority of the particles as spherical shaped ordered with twin boundaries and multiple facets. 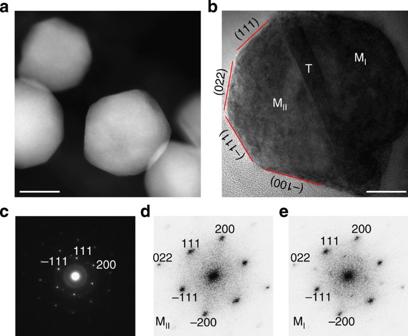Figure 4: Multiple facets of AuPdCo nanoparticles along with its selected-area electron diffraction patterns. (a,b) STEM and HRTEM image of AuPdCo-intermetallic nanoparticles showing multiple facets, respectively. Both scale bars, 10 nm. (c) EDP ofbas viewed along [0–11] direction. (d,e) The diffractograms from MIIand MI, respectively. Figure 4: Multiple facets of AuPdCo nanoparticles along with its selected-area electron diffraction patterns. ( a , b ) STEM and HRTEM image of AuPdCo-intermetallic nanoparticles showing multiple facets, respectively. Both scale bars, 10 nm. ( c ) EDP of b as viewed along [0–11] direction. ( d , e ) The diffractograms from M II and M I , respectively. Full size image Catalytic activity of AuPdCo nanostructures The polarization curves for the ORR obtained with Pt/C (3.5 nm), AuPdCo/C-core-shell and AuPdCo/C-intermetallic electrocatalysts as thin films on a rotating disk electrode (RDE) in an O 2 -saturated 0.1 M HClO 4 and 0.1 M KOH solution at 1,600 r.p.m. are shown in Fig. 5a,b , respectively. In acid electrolyte, as shown in Fig. 5a , AuPdCo/C-intermetallic and Pt/C have similar ORR onset potentials, whereas AuPdCo/C-core-shell electrocatalyst suffered a 40 mV loss. As illustrated in Fig. 5b , in alkaline solution also the AuPdCo/C-core-shell electrocatalyst suffered 15 mV loss in ORR onset potential compared with AuPdCo/C-intermetallic and Pt/C catalyst. In the region where the current approaches the mixed kinetic/diffusion regime, the half-wave potential measured to evaluate the electrocatalytic activity of the catalyst indicates that the intermetallic structure of AuPdCo/C catalyst increases the ORR activity almost comparable to Pt/C. Density functional theory studies have shown that the reactivity of the surface changes when Pd is alloyed with a 3d metal due to changes in its electronic structure, thus increasing the ORR activity [38] , [39] . The cyclic voltammograms (CV) recorded in Ar-saturated 0.1 M KOH solution at room temperature ( Supplementary Fig. 5 ) show that during the cathodic sweep, the peak for the reduction of Pd oxide appeared around 0.8 V for the AuPdCo/C-intermetallic nanoparticles, of which the peak position was a little positive to those of AuPdCo/C-core-shell nanoparticles, and even more positive than that of the commercial Pd/C catalysts. Similar observation was made in the CV recorded in Ar-saturated 0.1 M HClO 4 solutions. We envisage that the enhancement in the ORR kinetics of AuPdCo/C-intermetallic catalyst is due to changes in the electronic structure of surface Pd by the intermetallic ordering of atoms, together with the generation of smooth and low-index facets on the surfaces [40] , [41] . This increase in ORR activity when quantified by calculating the precious metal mass activity at 0.9 V (reversible hydrogen electrode (RHE)) is almost comparable to Pt/C ( Supplementary Table 1 ). But taking into account the material cost factor, the AuPdCo/C catalyst require cheaper Co-10 wt.%, Pd-8 wt.% and Au-2 wt.% to the Pt/C-20 wt.% metal catalyst, this intermetallic catalyst shows a significant economic importance. The results of the ORR catalysed by AuPdCo nanoparticles annealed at different temperatures are compiled in the Supplementary Table 1 . 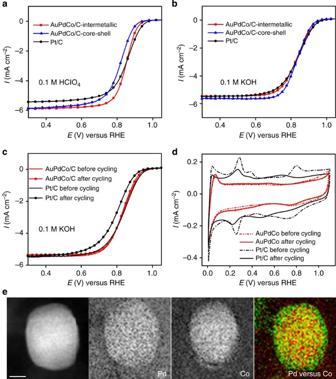Figure 5: ORR performance and structural stability of the catalyst. (a,b) ORR Polarization curves for AuPdCo/C- intermetallic and core-shell catalyst along with Pt/C catalyst on an RDE electrode in 0.1 M HClO4and 0.1 M KOH, respectively. Precious metal loading was 7.65 μg cm−2for AuPdCo catalysts and 6.0 μg cm−2for Pt catalyst. (c,d) ORR polarization and cyclic voltammetry curves of AuPdCo/C-intermetallic and Pt/C catalysts before and after 10,000 cycle test between 0.6 and 1.0 V in 0.1 M KOH. (e) HRTEM image of a single AuPdCo-intermetallic nanoparticle along with its EELS mapping and overlapped mapping (Pd (green) and Co (red)) showing the intermetallic structure of PdCo atoms after electrochemical cycling. Scale bar, 5 nm. Figure 5: ORR performance and structural stability of the catalyst. ( a , b ) ORR Polarization curves for AuPdCo/C- intermetallic and core-shell catalyst along with Pt/C catalyst on an RDE electrode in 0.1 M HClO 4 and 0.1 M KOH, respectively. Precious metal loading was 7.65 μg cm −2 for AuPdCo catalysts and 6.0 μg cm −2 for Pt catalyst. ( c , d ) ORR polarization and cyclic voltammetry curves of AuPdCo/C-intermetallic and Pt/C catalysts before and after 10,000 cycle test between 0.6 and 1.0 V in 0.1 M KOH. ( e ) HRTEM image of a single AuPdCo-intermetallic nanoparticle along with its EELS mapping and overlapped mapping (Pd (green) and Co (red)) showing the intermetallic structure of PdCo atoms after electrochemical cycling. Scale bar, 5 nm. Full size image The durability of the catalysts was evaluated by potential cycling between 0.5 and 1.00 V for 10,000 cycles in air-saturated 0.1 M KOH solution at a scan rate of 50 mV s −1 . The CV of the nanoparticles as shown in Fig. 5d obtained after 10,000 cycles show no change in the oxidation/reduction peaks indicating that the structure is intact. The core-shell-structured AuPdCo/C catalyst lost some of its electrochemical surface area as shown in the CV ( Supplementary Fig. 7 ) after 10,000 potential cycles. Pt/C catalyst too showed ( Fig. 5d ) some deterioration in the oxidation/reduction peaks which furthermore impacts the ORR activity. After 10,000 cycles, the Pt/C also revealed in previous studies [16] , results in the decaying of the redox peaks clearly indicating its poor stability. The ORR activity measured in terms of half-wave potential, as illustrated in Fig. 5c , decays ~30 mV for Pt/C, 19 mV for AuPdCo/C-core-shell catalysts ( Supplementary Fig. 7 ) after 10,000 electrochemical cycles whereas AuPdCo-intermetallic catalyst stays sturdy with no change in its half-wave potential. To get a better insight as to the particle size having an important role in the degradation mechanism, the intermetallic catalyst was compared with the Pt/C catalyst annealed using the same parameters of that of intermetallic nanoparticles. The high-temperature annealed Pt/C catalyst (9 nm particle size; Supplementary Fig. 12 ) suffered a loss of 18 mV in its half-wave potential after 10,000 cycles, concurrent with the previous reports [42] , [43] that larger particle size can reduce the rate of degradation. The structural stability of AuPdCo/C-intermetallic nanoparticles after electrochemical cycling was verified by ADF-STEM images and EELS elemental mapping as shown in Fig. 5e . Though the surface Co may have been leached away, the intermetallic structures of the PdCo nanoparticles along with surface Au atoms were preserved ( Supplementary Fig. 10 ). It’s for sure that the Au clusters on the surfaces promote the enhanced stability of this catalyst [36] , but the electronic effect due to the structural ordering and the formation of smooth, high-coordinated surfaces also contribute to the increase in the durability [40] . The durability of the AuPdCo-intermetallic catalyst for ORR in acid after 3,000 cycles ( Supplementary Fig. 8 ) showed a loss of 20% in ECSA and 45 mV decay in half-wave potential. In general intermetallic structures are more stable than their counterparts, but then the surface Pd might be leaching off creating vacancies further deteriorating the catalyst due to the harsh acid environment [15] . Further optimization of composition of the AuPdCo-intermetallic catalyst by varying the ratio of Au, Pd and Co precursors can provide an enhancement to the stability issues in acid media. In addition, these nanoparticles showed much better durability and activity in acid solution by using it as anode catalyst for fuel cells. The results show that the intermetallic nanoparticles behave just like Pt catalyst for the hydrogen oxidation reaction (HOR) in acid ( Supplementary Fig. 9 ). Even though the HOR activity trend is not reliable when based on the data obtained using a rotating disc electrode due to the fast kinetics of HOR on Pt and Pd electrodes [44] , [45] , we are using these results to show that intermetallic structures of AuPdCo catalyst can be used in much broader applications in heterogeneous catalysis. We demonstrate that addition of gold atoms can promote structural ordering of PdCo nanoparticles under elevated temperatures. The as-synthesized AuPdCo core-shell nanoparticles when heated at different temperatures tend to grow in particle size, but the intermetallic structure is formed only at 800 °C. The XRD patterns ( Supplementary Fig. 11 ), show that the core-shell nanoparticles heated at 700 °C tend to grow with no change in its peak positions as compared with the nanoparticles heated at 600 °C. A small XRD peak position at 2 θ angle of 43.8° near the pure Co-metal (111) reflections similar to the intermetallic nanoparticles may have been caused by the Co planes indicating that the core-shell structure of the AuPdCo particles is undone at 700 °C. So the core-shell structure of the particles remains intact up to 600 °C whereas at 700 °C the core-shell structure is undone forming random alloys and further increase in temperature leads to restructuring of ordered intermetallic alloys. Moreover on the basis of the PdCo binary alloy phase diagrams, Pd and Co forms random alloys at elevated temperatures, which lowers their activity and stability for ORR [29] , [46] , [47] , [48] . The ORR activity is also affected by the pH and leads to different mechanism in acid and alkaline media [49] . In acidic media, nanoparticle size effect has an important role in increasing the electrochemical surface area, thus increasing the catalytic activity, but in alkaline media, only negligible changes were due to nanoparticle size effects [50] , [51] . In summary, we establish an innovative but simple methodology for synthesizing structurally ordered AuPdCo-intermetallic nanoparticles. Evolution of ordered intermetallic PdCo nanoparticles from the random alloyed core-shell PdCo nanoparticles by adding Au atoms was justified using the STEM-EELS and electron diffraction techniques. AuPdCo nanoparticles are a promising Pt-free catalyst with much intricacy of its electrochemical activity dependence on the structural ordering of its atoms. AuPdCo-intermetallic nanocatalyst shows comparable ORR activity with commercial Pt/C but much better long-term stability in alkaline medium. Since we use a simple and cost effective strategy to make structurally ordered intermetallic PdCo nanoparticles, it is believed that this approach may offer numerous possibilities in tailoring other transition metal intermetallics. Synthesis Carbon-supported AuPdCo nanoparticles was prepared by first mixing Vulcan carbon XC72R with CoCl 2 .6H 2 O salt in aqueous solution. Later, trisodium citrate dihydrate at a ratio of 1:3 with respect to Co salt was mixed with the carbon mixture while simultaneously purging the mixture with Ar under an ultrasonic bath for an hour. The Co salt was then reduced by adding NaBH 4 while simultaneously purging the mixture with Ar. After 5 min of reaction time, Pd(NO 3 ) 2 H 2 O and HAuCl 4 H 2 O salt mixture was added to the Co carbon mixture and sonicated for an hour so as to obtain AuPdCo core-shell nanoparticles. The final mixture obtained was washed and rinsed with Millipore water, and then dried. The nanoparticles obtained had a core-shell structure with mole fraction of Au 10 Pd 40 Co 50 . The as-prepared AuPdCo/C catalysts were annealed at 500 and 800 °C in H 2 stream for 30 min in a tube furnace. The latter temperature helped to obtain an atomic structure ordering of the nanoparticles while the former preserved the core-shell structure. Electrochemical testing Electrochemical measurements were conducted using the RDE setup with a potentiostat (CHI 700B potentiostat (CH Instruments)). Catalyst ink was prepared by ultrasonic mixing of 5 mg of catalyst in 5 ml of H 2 O. The catalyst ink of 10–15 μl was dropped on the glassy carbon substrate of the RDE electrode (5 mm in diameter, 0.196 cm 2 ). After drying in air, the electrode was covered with 10 μl of H 2 O diluted Nafion solution (2 μg per 5 μl) and dried again. All electrochemical measurements were carried out in an Ar-purged 0.1 M KOH/0.1 M HClO 4 aqueous solution using a three-electrode cell with a Pt wire as the counter electrode and a leak-free reference electrode (Ag/AgCl). All the potentials are reported with respect to RHE. The electrolytes were prepared from potassium hydroxide solution (Fluka) and perchloric acid (Fisher scientific), and MilliQ UV-plus water. Polarization curve for the ORR was obtained in O 2 -saturated solution by scanning the potential from 0 to 1.1 V versus RHE (scan rate: 10 mV s −1 ; rotation rate: 225, 400, 625, 900, 1,225, 1,600 and 2,025 r.p.m.). For calculating the activity of the catalysts, the kinetic currents for ORR were determined using the Koutecky–Levich equation [14] , [52] ( Supplementary Fig. 6 ). Characterization Synchrotron XRD measurements were carried out at National Synchrotron Light Source (NSLS), Brookhaven National Laboratory (BNL) using X18A beamline. The wavelength of X-ray used was 1.0 Å. Rigaku Ultima diffractometer using Cu Kα radiation (1.54056 Å) was used for other XRD patterns. STEM and EELS studies were conducted on the catalyst using Hitachi (HD-2700C) aberration-corrected STEM at the Center for Functional Nanomaterials (CFN), BNL. A 1.4 Å electron probe with probe current ~50 pA and an electron source with energy resolution of 0.35 eV were used in this study. The microscope was equipped with a cold field emission electron source and a high-resolution Gatan Enfina energy-loss spectrometer. Element-sensitive EELS mapping was carried out for Au M-edge, Pd M-edge and Co L-edge across single solid particles. HRTEM and electron diffraction analysis were carried out using the JEM-ARM200F microscope equipped with cold field emission gun and double aberration correctors at the accelerating voltage of 200 kV. The HRTEM image and diffractograms were simulated using our own computer codes based on the multislice method [53] . The calculated images were convoluted with a 0.06 nm FWHM Gaussian spread function to compare with the experiments. The fcc structure can be also described by a hexagonal lattice with a h =1/√2 a c and c h =√3 a c , where a h and c h , and a c denote the lattice parameters of hexagonal lattice and fcc lattice, respectively. The relationship between the fcc and hexagonal lattice: (111) c ||(001) h ( Supplementary Fig. 4 ). How to cite this article : Kuttiyiel, K. A. et al . Gold-promoted structurally ordered intermetallic palladium cobalt nanoparticles for the oxygen reduction reaction. Nat. Commun. 5:5185 doi: 10.1038/ncomms6185 (2014).